Large orbital polarization in nickelate-cuprate heterostructures by dimensional control of oxygen coordination 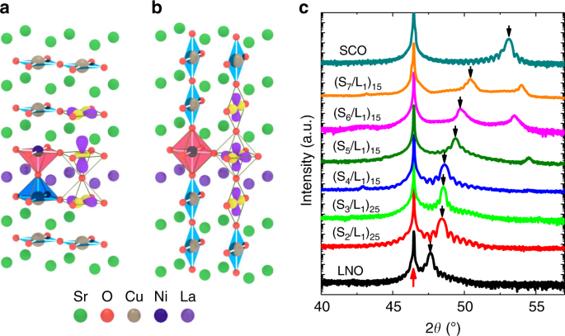Fig. 1 Interfacial engineering of oxygen coordination in SrCuO2/LaNiO3superlattices. Schematics for SrCuO2/LaNiO3(SCO/LNO) heterostructures withaplanar-type SrCuO2andbchain-type SrCuO2, resulting in different oxygen coordination and orbital polarization of Ni ions in LaNiO3.cX-ray diffraction (XRD)θ–2θscans of a LaNiO3film (34 nm in thickness), ((SrCuO2)N/(LaNiO3)1)M(noted as (SN/L1)M) superlattices, and a SrCuO2film (28 nm). The red and black arrows indicate the SrTiO3002 peak and the peaks from superlattices or films, respectively, showing a clear modulation of out-of-plane lattice constants Artificial heterostructures composed of dissimilar transition metal oxides provide unprecedented opportunities to create remarkable physical phenomena. Here, we report a means to deliberately control the orbital polarization in LaNiO 3 (LNO) through interfacing with SrCuO 2 (SCO), which has an infinite-layer structure for CuO 2 . Dimensional control of SCO results in a planar-type (P–SCO) to chain-type (C–SCO) structure transition depending on the SCO thickness. This transition is exploited to induce either a NiO 5 pyramidal or a NiO 6 octahedral structure at the SCO/LNO interface. Consequently, a large change in the Ni d orbital occupation up to ~30% is achieved in P–SCO/LNO superlattices, whereas the Ni e g orbital splitting is negligible in C–SCO/LNO superlattices. The engineered oxygen coordination triggers a metal-to-insulator transition in SCO/LNO superlattices. Our results demonstrate that interfacial oxygen coordination engineering provides an effective means to manipulate the orbital configuration and associated physical properties, paving a pathway towards the advancement of oxide electronics. The correlated d -orbital plays a central role in creating collective phenomena in transition metal oxides, since the s -electrons of transition metals are transferred to oxygen ions, and the remaining d -electrons determine the delicate interplay between spin, charge, and orbital degrees of freedom [1] . For example, superexchange can induce either antiferromagnetic or ferromagnetic coupling of spins depending on the orbital filling and ordering, yielding a vast array of magnetic ground states [2] , [3] , [4] , [5] . In high transition temperature ( T C ) cuprate superconductors, the x 2 − y 2 orbital character is crucial for Cooper pairing [6] . The remarkable Mott metal-insulator transition often found in correlated oxides can be engineered by tailoring the orbital occupancy [7] . Thus, identifying ways to deliberately control the orbital degree of freedom in correlated oxides is highly desirable to discover electronic and magnetic phenomena that are useful for developing oxide electronic and spintronic devices. Interface engineering is a powerful method to manipulate such orbital degrees of freedom [7] , [8] , [9] , [10] , [11] , [12] , [13] and has revealed many intriguing phenomena not possible in bulk material counterparts, such as interfacial charge transfer, orbital covalency, and broken inversion symmetry at nanometer scale [12] , [13] , [14] , [15] , [16] , [17] , [18] , [19] . Rare-earth nickelate (RNiO 3 ) heterostructures provide good experimental and theoretical frameworks to investigate influence of orbital occupation on the physical properties [17] , [18] , [19] , [20] , [21] , [22] , [23] , [24] . The d 7 ionic configuration of Ni 3+ in nickelates contains a full t 2g shell and a single electron occupying the e g orbital. This orbital configuration generally favors a Jahn–Teller distortion as observed in LaMnO 3 [25] . However, the e g orbitals in nickelates are doubly degenerate. A recent theoretical study proposed that the planar x 2 -y 2 orbital order could be realized by spatially confining LaNiO 3 into a ultrathin layer between two insulators, leading to a cuprate-like Fermi surface and, subsequently, high T C superconductivity [23] , [24] . This idea triggered enormous experimental efforts to study the RNiO 3 systems. However the orbital polarization caused by spatial confinement and strain was much smaller than the predicted one [17] , [26] , [27] , [28] . 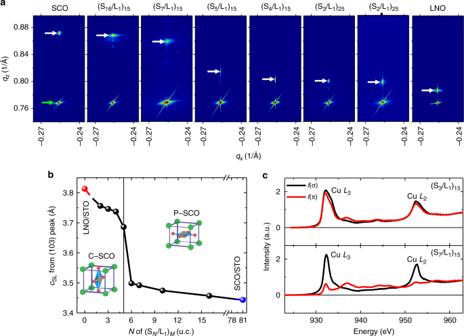Fig. 2 Dimensional control of the sub-lattice structure of SrCuO2.aReciprocal space mapping of the 103 peak of a LaNiO3(LNO) film, ((SrCuO2)N/LNO1)Msuperlattices and a SrCuO2(SCO) film. The green and white arrows indicate SrTiO3(STO) substrate and film/superlattice peaks, respectively.bOut-of-plane lattice constant (c) as a function SCO sublayer thickness (N). The sudden change ofcacrossN= 5 u.c. indicates a structural transition from a planar type to a chain type.cPolarization dependent XAS of CuL2,3edge for S7/L1(top panel) and S3/L1(bottom panel) superlattices, demonstrating a clear contrast on the orbital population Resonant inelastic X-ray scattering indicated a very minor e g splitting energy \(( {\Delta E_{e_{\mathrm{g}}}} )\) induced by heterostructural engineering [29] . It has also been suggested that nickelate thin films prefer to retain their preferred electronic and structural configurations determined by the bulk phase, which limits the control of the orbital parameters through heterostructural engineering [30] . Here, we report that one can largely manipulate the occupancy of Ni 3 d orbitals in LNO-SrCuO 2 (SCO) heterostructures by dimensional control of the SCO layers. The SCO which in the bulk phase is orthorhombic (Cmcm) with a double-chain structure formed in a perovskite like framework with missing apical oxygen in thin films [31] , [32] . Upon reducing the thickness when grown in thin films, the planar-type structure of SCO (P–SCO) is transformed to a chain-type structure (C–SCO) [33] , [34] , [35] . The CuO 2 planes of P–SCO and C–SCO are parallel and perpendicular with respect to the film plane, respectively. This difference effectively yields two different heterostructures (see Fig. 1a, b ). In the case of a P–SCO/LNO heterostructure grown on a B-site terminated ABO 3 perovskite substrate, the interfacial atomic stacking sequence is hypothesized to be (CuO 2 /Sr)/(NiO 2 /LaO), leading to a truncated NiO 5 pyramid structure (see Fig. 1a ). On the other hand, the stacking sequence for the C–SCO/LNO interface would become (CuO/SrO)/(NiO 2 /LaO), which yields an octahedrally coordinated Ni and thus no modification of the LNO structure (see Fig. 1b ). Our results demonstrate how the unique infinite-layer structure offered in SCO can be utilized to induce a very large Ni 3 d orbital polarization in P–SCO/LNO superlattices or to create degenerate (i.e., little or no polarization) Ni e g orbitals in C–SCO/LNO superlattices as sketched in Fig. 1a, b . The observed changes in the electronic and orbital states may have a profound impact on transport properties of SCO/LNO superlattices. Fig. 1 Interfacial engineering of oxygen coordination in SrCuO 2 /LaNiO 3 superlattices. Schematics for SrCuO 2 /LaNiO 3 (SCO/LNO) heterostructures with a planar-type SrCuO 2 and b chain-type SrCuO 2 , resulting in different oxygen coordination and orbital polarization of Ni ions in LaNiO 3 . c X-ray diffraction (XRD) θ –2 θ scans of a LaNiO 3 film (34 nm in thickness), ((SrCuO 2 ) N /(LaNiO 3 ) 1 ) M (noted as (S N /L 1 ) M ) superlattices, and a SrCuO 2 film (28 nm). The red and black arrows indicate the SrTiO 3 002 peak and the peaks from superlattices or films, respectively, showing a clear modulation of out-of-plane lattice constants Full size image Dimensional control of the sub-lattice structure of SrCuO 2 LNO and SCO films and their superlattices were grown on TiO 2 terminated (001) SrTiO 3 (STO) substrates by pulsed laser epitaxy. The growth condition was optimized to achieve high-quality SCO films in the bulk planar structure (see Supplementary Fig. 1 ), and all films were atomically flat with step-terrace features on their surfaces (See Supplementary Fig. 2 ). As shown in Fig. 1c , X-ray diffraction (XRD) θ –2 θ scans of an 80 unit-cell (u.c.) SCO film revealed clearly the SCO 002 peak near 2 θ = 53 o , confirming the bulk-like infinite-layer structure [33] , [34] . Using the same growth conditions, high-quality LNO films were obtained as well. When growing (SCO N /LNO 1 ) M superlattices (noted as S N /L 1 ), a systematic change in XRD spectra was observed with increasing the SCO layer thickness. Since the P–SCO and C–SCO have quite different out-of-plane lattice constants of ~3.45 Å (2 θ = 53 o ) and ~3.8 Å (2 θ = 47.8 o ), respectively [33] , [35] , the position of the main superlattice peak SL(0) can be used to identify the SCO structure type. For relatively thick SCO layers (e.g., N = 7 u.c. ), SL(0) was located between the SCO 002 and the LNO 002 XRD peaks, suggesting the formation of the planar-type SCO structure within the superlattice. When the SCO layer thickness is reduced to 2 u.c., the SL(0) peak shifts close to the LNO 002 peak, indicating that 2 u.c.-thick SCO has a similar out-of-plane lattice constant with that of LNO. This result suggests that a chain-type SCO structure was formed in the S 2 /L 1 superlattice. With increasing the SCO film thickness to 5 u.c., a sudden large shift of the superlattice peaks occurred. This shift suggests the critical thickness of the phase conversion from P–SCO to C–SCO to be at 5 u.c.. This thickness-driven transition of the SCO structure in SCO/LNO superlattices was also observed for other LNO sublayer thicknesses (see Supplementary Fig. 3 ). Further evidence of the structural transition triggered by reducing the SCO thickness was observed from XRD reciprocal space mapping (RSM). The RSM shown in Fig. 2a indicates that all the superlattices and reference SCO and LNO films were coherently grown on STO substrates. The reciprocal lattice vector ( q z ) of thick SCO superlattices (e.g., N = 7 and 16 in S N /L 1 ) was very close to that of a P–SCO film, confirming that the SCO layers in the superlattices possess the bulk-like planar-type structure. On the other hand, the q z of thin SCO superlattices ( N = 2–4) was similar to that of a LNO film. Interestingly, as shown in Fig. 2b , the SCO thickness dependent change in the out-of-plane lattice constant ( c SL ) calculated from the RSMs around the 103 peak ( c SL = 3/ q z ) clearly reveals a sudden transition at around 5 u.c. of the SCO sublayer thickness. If the bulk-like P–SCO is maintained when the SCO thickness is reduced, one can only expect a gradual increase in c SL . Therefore, our observation of the step-like transition shown in Fig. 2a, b unambiguously demonstrates that the planar-type lattice structure of SCO can be converted into the chain-type structure by reducing the SCO thickness below 5 u.c. Detailed XRD and transport analyses further suggest the formation of a twin domain structure within the chain-type SCO (see supplementary Fig. 4 ), originating from the two-fold symmetry of C–SCO on the four-fold (001) STO substrate. Fig. 2 Dimensional control of the sub-lattice structure of SrCuO 2 . a Reciprocal space mapping of the 103 peak of a LaNiO 3 (LNO) film, ((SrCuO 2 ) N /LNO 1 ) M superlattices and a SrCuO 2 (SCO) film. The green and white arrows indicate SrTiO 3 (STO) substrate and film/superlattice peaks, respectively. b Out-of-plane lattice constant ( c ) as a function SCO sublayer thickness ( N ). The sudden change of c across N = 5 u.c. indicates a structural transition from a planar type to a chain type. c Polarization dependent XAS of Cu L 2,3 edge for S 7 /L 1 (top panel) and S 3 /L 1 (bottom panel) superlattices, demonstrating a clear contrast on the orbital population Full size image Such a change in the orientation of the oxygen plane can be confirmed as a change in the orbital occupancy measured from linearly polarized X-ray absorption spectroscopy (XAS) acquired in fluorescence yield (FY) mode. The orbital occupancy of Cu x 2 - y 2 and 3z 2 -r 2 orbitals was probed by the XAS measured with in-plane (σ) and out-of-plane (π) polarized x-rays, respectively. As shown in Fig. 2c , the large I (σ) versus I (π) XAS of the Cu L 2,3 -edge of the S 7 /L 1 superlattice indicates exclusive \(3d_{x^2 - y^2}\) character, consistent with orbital configuration in layer-structured cuprates (see supplementary Fig. 5 ). By contrast, I (σ) and I (π) share a similar intensity and shape for the S 3 /L 1 superlattice, suggesting the chain-type SCO structure and \(3d_{y^2 - z^2}\) orbital character [36] . Additionally, the change in the SCO microstructure and oxygen coordination of Ni were confirmed by scanning transmission electron microscopy (STEM) (see Supplementary Fig. 6 ), consistent with XRD and XAS data. Engineered Ni orbital polarization in SrCuO 2 -LaNiO 3 superlattices Now we turn to investigate the reconstruction of the Ni e g orbital. 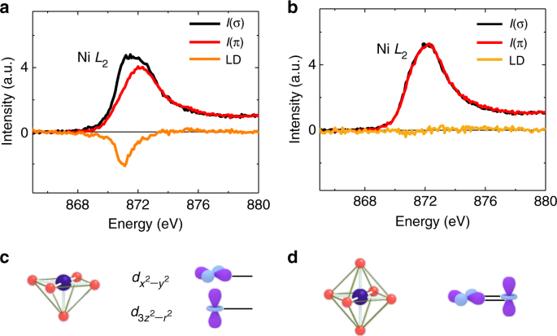Fig. 3 Orbital polarization of the Ni-3dorbital by oxygen coordination control.aPolarization dependent X-ray absorption spectroscopy (XAS) of NiL2edge foraS7/L1andbS3/L1superlattices. Large linear dichroism (LD) is observed for the S7/L1SL, whereas the LD is nearly zero for the S3/L1SL. Schematics of theegorbital configuration are shown forcS7/L1anddS3/L1superlattices Figure 3a shows the XAS of the Ni L 2 -edge of an S 7 /L 1 superlattice. 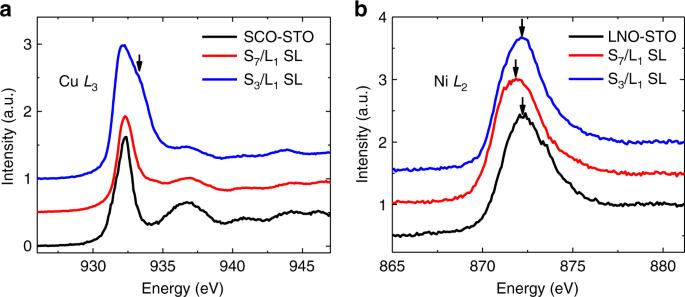Fig. 4 The charge states of Cu and Ni in different superlattices.aX-ray absorption spectroscopy (XAS) of CuL3-edge for a SrCuO2(SCO) film and (SCO7/(LaNiO3)1) (noted as S7/L1) and S3/L1superlattices (SL). A shoulder indicated by the black arrow arises from Cu d9Lstate.bXAS of NiL2-edge for a LaNiO3(LNO) film and S7/L1and S3/L1superlattices. A slight shift of the peak position to a lower energy for S7/L1superlattice suggests an electron doping in the LNO layer. The XAS is obtained by averaging linearly polarized XAS (I= (I(σ) +I(π))/2) Since the Ni L 3 -edge largely overlaps with the La M -edge, and FY of the La 3+ (4 f 0 ) M -edge deviates from the true XAS for the conventional detection geometry used, the Ni L 2 -edge is more suitable to illustrate the orbital reconstruction (see supplementary Fig. 7 ) [17] . The I (σ) exhibits a higher intensity than I (π), indicating that holes prefer to occupy the \(3d_{x^2 - y^2}\) orbital. For the S 3 /L 1 superlattice, the I (σ) and I (π) intensities are similar to each other. Therefore, the Ni e g orbital is degenerate (Fig. 3b ). The different orbital configuration between the S 7 /L 1 superlattice and the S 3 /L 1 superlattice is also observed in total electron yield mode (see supplementary Fig. 7 ), indicating that the observed polarization dependence of the FY XAS originates from the intrinsic orbital polarization. The orbital configuration in the S 3 /L 1 superlattice confirms the chain-type SCO structure within the S 3 /L 1 superlattice, which recovers the octahedral coordination. Using the difference between in-plane polarized absorption I ( ab ) and out-of-plane polarized absorption I ( c ), the ratio of unoccupied states, r , can be quantified using the following sum rule [17] , [37] 
    r = h_3z^2 - r^2/h_x^2 - y^2 = 3I(c)/4I(ab) - I(c)
 (1) Fig. 3 Orbital polarization of the Ni-3 d orbital by oxygen coordination control. a Polarization dependent X-ray absorption spectroscopy (XAS) of Ni L 2 edge for a S 7 /L 1 and b S 3 /L 1 superlattices. Large linear dichroism (LD) is observed for the S 7 /L 1 SL, whereas the LD is nearly zero for the S 3 /L 1 SL. Schematics of the e g orbital configuration are shown for c S 7 /L 1 and d S 3 /L 1 superlattices Full size image Here, a , b , and c are the Cartesian coordination axis of the substrates with c along out-of-plane direction and h is the hole occupancy. The π-polarized absorption I (π) was corrected for the angle θ = 20 o between the incident X-rays and sample plane in our experimental setup using I ( c ) = [ I (π) − I ( ab )sin 2 θ ]/cos 2 θ , while the orientation of the incident beam with respect to the sample did not affect I (σ) and I ( ab ) = I (σ). The linear dichroism (LD) [ LD = I ( c ) − I ( ab )] shown in Fig. 3a, b further emphasizes the orbital polarization of the S 7 /L 1 superlattice. Using the integrated intensity of I ( ab ) and I ( c ) from background-subtracted XAS, the hole ratio r can be quantified (see supplementary Fig. 8 ). The r values for S 7 /L 1 and S 3 /L 1 superlattices are 0.7 and 1.0, respectively, suggesting a predominant x 2 − y 2 hole character in S 7 /L 1 and degenerate orbital in S 3 /L 1 . Previously, the r value of the largest orbital polarization \([ {P = ( {n_{x^2 - y^2} - n_{3z^2 - r^2}} )/( {n_{x^2 - y^2} + n_{3z^2 - r^2}} )} ]\) achieved by inducing tensile strain was ~1.19 [26] . The spatial confinement in LAO/LNO superlattices has been reported to result in a value of r ~ 1.05 [17] , [27] . The hole ratio that we observed cannot be compared directly to these previous values since our experiments had a flipping orbital configuration in which the \(3d_{3z^2 - r^2}\) orbital has more hole occupancy. The relative change of occupancy (≡|1 − r |) is instead used here for a quantitative comparison. In comparison to ~19% by strain [26] and ~5% by spatial confinement [17] , [27] , the observed 30% change of Ni orbital occupancy in P–SCO/LNO superlattice confirms the significant impact of oxygen coordination on orbital reconstruction. The prevailing \(3d_{x^2 - y^2}\) character cannot be explained by spatial confinement, which favors the \(3d_{3z^2 - r^2}\) hole occupancy due to the confinement of the \(3d_{3z^2 - r^2}\) orbital in the z direction [17] , [23] , [24] , [38] . We attribute the observed large orbital polarization in the S 7 /L 1 superlattice to the NiO 5 pyramid structure, which is expected to lower the \(3d_{3z^2 - r^2}\) with respect to \(3d_{x^2 - y^2}\) [39] . In fact, our polarization dependent XAS revealed quite similar features to the square-planar La 4 Ni 3 O 8 and YBa 2 Cu 3 O 7 (YBCO) single crystals [36] , [40] . The La 4 Ni 3 O 8 is comprised of NiO 2 planar structures while the main building block of YBCO is a CuO 5 pyramid [40] , [41] . These two materials possess similar e g band structures with the \(3d_{3z^2 - r^2}\) lying lower than \(3d_{x^2 - y^2}\) . In sharp contrast, there is a negligible orbital polarization when the apical oxygen is retained in the S 3 /L 1 superlattice. Although there is still tensile strain on LNO within the S 3 /L 1 superlattice, the observed degenerate e g orbital indicates that the octahedrally coordinated Ni prefers to retain a bulk-like electronic configuration. This retainment of bulk orbital configuration was reported previously [30] and is also observed in our LNO films (see Supplementary Fig. 9 ). The corresponding e g orbital energy diagrams for the NiO 5 pyramid and the NiO 6 octahedron are schematically plotted in Fig. 3c (S 7 /L 1 ) and Fig. 3d (S 3 /L 1 ). Using the outermost filled orbital, a sketch of the orbital configuration in SCO/LNO superlattice is plotted Fig. 1a, b , demonstrating the designed orbital configuration through heterostructural engineering. The charge states of Cu and Ni at interfaces The charge states of Cu and Ni are further investigated using XAS. As shown in Fig. 4a , the Cu L -edge spectrum of a S 7 /L 1 superlattice shows a characteristic Cu 2+ feature as observed in SCO films [36] , [42] . Meanwhile, the S 3 /L 1 superlattice shows a strong shoulder at ~933.28 eV, which is positioned ~1 eV higher than that of the Cu 2+ peak and is consistent with the d 9 L state [36] , [42] . Here L represents the ligand hole. The doped holes are unlikely from interfacial charge transfer, since the Ni in S 3 /L 1 maintains Ni 3+ as demonstrated by the lack of Ni L -edge shift (see Fig. 4b ). Further, La interdiffusion should favor Cu 1+ . It is more likely that the hole arises from oxygen excess SrCuO 2+ x . For the S 7 /L 1 superlattice, the Ni L -edge shifts by about −0.3 eV relative to that of the LNO film. Since a 1 eV shift corresponds to roughly one electron valence change [43] , [44] , the energy shift suggests an averaged Ni 2.7+ valence state in S 7 /L 1 . It has been reported that doped electrons at a LNO/La 2 CuO 4 interface are predominantly accommodated by change of Ni valence [45] . A similar situation may occur for a SCO/LNO interface where a possible formation of oxygen vacancies may dope the interface state with electrons. Fig. 4 The charge states of Cu and Ni in different superlattices. a X-ray absorption spectroscopy (XAS) of Cu L 3 -edge for a SrCuO 2 (SCO) film and (SCO 7 /(LaNiO 3 ) 1 ) (noted as S 7 /L 1 ) and S 3 /L 1 superlattices (SL). A shoulder indicated by the black arrow arises from Cu d 9 L state. b XAS of Ni L 2 -edge for a LaNiO 3 (LNO) film and S 7 /L 1 and S 3 /L 1 superlattices. A slight shift of the peak position to a lower energy for S 7 /L 1 superlattice suggests an electron doping in the LNO layer. The XAS is obtained by averaging linearly polarized XAS ( I = ( I (σ) + I (π))/2) Full size image Controlled metal-to-insulator transition Functionally, we see that these observed changes to electronic and orbital states have a profound impact on transport properties of SCO/LNO superlattices. 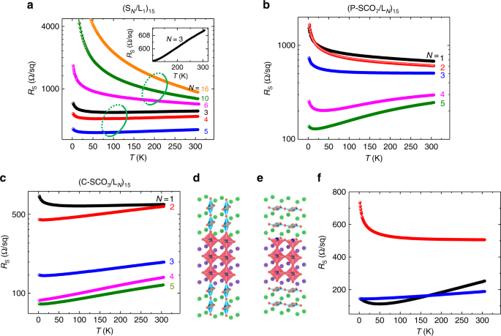Fig. 5 Metal-to-insulator transition by dimensionality control in superlattices. Temperature dependent sheet resistance ofa(SN/L1)15,b(P–SCO7/LN)15, andc(C–SCO3/LN)15for various layer thickness (N) ofaSCO orb,cLNO. The green ellipses inagroup separately the metallic and insulating superlattices. S, L, P–SCO, and C–SCO represent SrCuO2(SCO), LaNiO3(LNO), planar-type SCO, and chain-type SCO, respectively. Structural models ford(C–SCO7/L3)15ande(P–SCO3/L3)15superlattices.fTemperature dependent sheet resistance of (C–SCO7/L3)15(blue curves), (P–SCO3/L3)15(red curves), and (STO7/L3)15(black curves). The transport properties illustrate a metal-to-insulator transition in 3 u.c. LNO layer when the top surface is transformed from the octahedral coordination to the pyramidal coordination Figure 5a shows the transport properties of S N /L 1 superlattices with different SCO thicknesses. The S N /L 1 superlattices exhibit a metallic behavior (d R /d T > 0) to insulating behavior (d R /d T < 0) transition (MIT) with increasing the SCO layer thickness. The critical thickness for MIT is 5 u.c., which coincides with the critical thickness for a structural transition (see Fig. 2 ). This fact suggests that the P–SCO N /LNO 1 and C–SCO N /LNO 1 superlattices are insulating and metallic, respectively. Since LNO will undergo a MIT with reducing thickness across ~3–5 u.c. [46] , [47] , [48] , [49] , the single unit-cell LNO should be insulating and thus the metallic behavior arises from the C–SCO layer, which can be explained by the hole doping as observed by XAS (see Fig. 4a ). Fig. 5 Metal-to-insulator transition by dimensionality control in superlattices. Temperature dependent sheet resistance of a (S N /L 1 ) 15 , b (P–SCO 7 /L N ) 15 , and c (C–SCO 3 /L N ) 15 for various layer thickness ( N ) of a SCO or b , c LNO. The green ellipses in a group separately the metallic and insulating superlattices. S, L, P–SCO, and C–SCO represent SrCuO 2 (SCO), LaNiO 3 (LNO), planar-type SCO, and chain-type SCO, respectively. Structural models for d (C–SCO 7 /L 3 ) 15 and e (P–SCO 3 /L 3 ) 15 superlattices. f Temperature dependent sheet resistance of (C–SCO 7 /L 3 ) 15 (blue curves), (P–SCO 3 /L 3 ) 15 (red curves), and (STO 7 /L 3 ) 15 (black curves). The transport properties illustrate a metal-to-insulator transition in 3 u.c. LNO layer when the top surface is transformed from the octahedral coordination to the pyramidal coordination Full size image Figure 5b, c show the LNO layer thickness dependent transport properties in P–SCO 7 /L N and C–SCO 3 /L N superlattices, respectively. With reducing thickness of LNO layers, the P–SCO 7 /L N superlattices gradually evolve from a metallic state to an insulating state. Such behavior is similar to MIT in single LNO films, which is associated with dimensional crossover [46] , [49] . What is more, the 3 u.c. critical thickness for MIT in P–SCO 7 /L N is also similar to bare LNO films [46] , [47] , [48] , [49] . These results strongly suggest that the MIT in P–SCO 7 /L N is driven by LNO sub-layers. Since the C–SCO is metallic, all C–SCO 3 /L N superlattices exhibit good metallic behavior regardless of the thickness of LNO (see Fig. 5c ). However, there is still a sharp decrease of the resistance when the LNO thickness is reduced from N = 3 to 2 u.c., while the C–SCO 3 /L 1 and C–SCO 3 /L 2 showed similar resistance values. This result implies a MIT in the LNO layers when reducing LNO thickness from 3 to 2 u.c. The different critical thickness ( t c ) for MIT of LNO in P–SCO 7 /L N ( t c = 3) and in C–SCO 3 /L N ( t c = 2) indicates that a MIT in 3 u.c. LNO sublayer occurs when the top surface of the LNO layer is transformed from the octahedral coordination to the pyramidal coordination (Fig. 5d , e). This result is further emphasized by comparing the resistance of P–SCO 7 /L 3 with C–SCO 7 /L 3 superlattices in Fig. 5f . Although the metallic C–SCO layer also contributes to the transport, the transport behavior of C–SCO 3 /L 3 is dominated by the LNO layer since the resistance of C–SCO 3 /L 1 is ~2 times larger than that of C–SCO 3 /L 3 . To further confirm the effect of oxygen coordination on transport, we measured the transport properties of STO 7 /L N superlattices where the LNO interface has the same octahedral coordination as that in C–SCO 3 /L 3 . The critical thickness for MIT in STO 7 /L N is 2 u.c. (see Supplementary Fig. 10 ), which is the same with C–SCO 3 /L N superlattices and thinner than P–SCO 7 /L N superlattices. This indicates that recovering the top pyramid NiO 5 in P–SCO 7 /L 3 to a full octahedral structure in STO 7 /L 3 or C–SCO 3 /L 3 will drive the LNO layer to be metallic. As shown in Fig. 5f , the STO 7 /L 3 is metallic and has a similar resistance with C–SCO 3 /L 3 . The relative small change of resistance from P–SCO 7 /L 3 to STO 7 /L 3 is due to the crossover MIT in LNO and also the fact that P–SCO is not a good insulator and contributes to the transport as well. Higher LNO resistance in P–SCO/LNO superlattices could be due to the reduced oxygen coordination, as observed in bare LNO films [50] , [51] . The smaller Ni e g bandwidth in pyramidal coordination and reduced in-plane electron hopping strength due to preferential 3 z 2 - r 2 orbital occupation would increase the resistance. Further, the appearance of Ni 2+ may also play a role by opening a charge excitation gap [38] , [43] . In conclusion, we have demonstrated that the orbital polarization and transport properties of SCO/LNO superlattices can be manipulated by templating the infinite structure of SCO into LNO through dimensionally controlling the oxygen coordination. Reducing the SCO thickness below 5 u.c. resulted in a structural transition from a planar-type to a chain-type structure. At SCO/LNO interfaces, the planar-type SCO structure induced a NiO 5 pyramidal structure in LNO, whereas the chain-type SCO structure yielded a NiO 6 octahedron in LNO, allowing us to selectively control the out-of-plane and in-plane orbital occupancies. This type of oxygen coordination manipulation could enhance the Ni orbital polarization up to ~30%. This enhancement is larger than that achieved from other means, including by strain (~19%) or spatial confinement (~5%). Our findings unambiguously demonstrate how the interfacial oxygen coordination engineering can effectively manipulate the orbital configuration and electronic properties, providing a possible new approach to realizing superconducting nickelates with high T c . The oxygen coordination control using SCO as a template could also be applied to other perovskites to explore previously inaccessible orbital-driven phenomena. Sample growth All superlattices and thin films were grown on TiO 2 terminated (001) SrTiO 3 substrates by pulsed laser epitaxy using a KrF excimer laser ( λ = 248 nm). The single TiO 2 terminated and atomically flat SrTiO 3 substrates were obtained by the etching with standard buffered-HF and subsequent annealing at 950 o C for 1.5 h. The laser fluence and repetition rate were fixed at 2 J cm −2 and 5 Hz, respectively. The oxygen partial pressure and substrate temperature were maintained at 100–150 mTorr and 650 o C, respectively. Sample characterization The surface morphology was characterized by atomic force microscopy. The lattice structure was characterized by a high-resolution four-circle X-ray diffractometer. Transport measurements were performed in a van-der-Pauw geometry using a Physical Property Measurement System. The TEY and FY XAS measurements of the Cu and Ni edges were performed at the beamline 4–ID–C of the Advanced Photon Source. XAS was measured at 300 K, with the X-rays at a grazing (20°) angle to the films surface, and the TFY detector at 90° from the incoming X-rays.